Oscillation of p38 activity controls efficient pro-inflammatory gene expression The p38 MAP kinase signalling pathway controls inflammatory responses and is an important target of anti-inflammatory drugs. Although pro-inflammatory cytokines such as interleukin-1β (IL-1β) appear to induce only transient activation of p38 (over ∼ 60 min), longer cytokine exposure is necessary to induce p38-dependent effector genes. Here we study the dynamics of p38 activation in individual cells using a Förster resonance energy transfer (FRET)-based p38 activity reporter. We find that, after an initial burst of activity, p38 MAPK activity subsequently oscillates for more than 8 h under continuous IL-1β stimulation. However, as this oscillation is asynchronous, the measured p38 activity population average is only slightly higher than basal level. Mathematical modelling, which we have experimentally verified, indicates that the asynchronous oscillation of p38 is generated through a negative feedback loop involving the dual-specificity phosphatase MKP-1/DUSP1. We find that the oscillatory p38 activity is necessary for efficient expression of pro-inflammatory genes such as IL-6 , IL-8 and COX-2 . Mitogen-activated protein kinases (MAPKs) constitute major signalling pathways through which eukaryotic cells respond to extracellular stimuli [1] , [2] . There are several subfamilies of MAPKs in higher eukaryotes, including extracellular signal-regulated kinase (ERK), c-Jun amino-terminal kinase (JNK) and p38 MAPK (p38). All MAPKs are activated through a three-tiered kinase cascade, composed of an MAPK, an MAPK kinase (MAPKK) and a MAPKK kinase (MAPKKK). Distinct MAPKKKs activated by a specific stimulus phosphorylate and thereby activate a cognate MAPKK, which then phosphorylates and activates a downstream MAPK. The ERK MAPKs are activated by various growth factors and control cell growth and proliferation. In contrast, the p38 and JNK MAPKs are activated by stress conditions, including ultraviolet, oxidative stress and inhibition of protein synthesis by antibiotics such as anisomycin [3] . In general, if the intensity of the stress is moderate, the affected cell will seek to repair the damage. If, however, the stress is too severe for a complete repair, the affected cells are eliminated by apoptosis. For example, sustained activation of p38 and JNK, and concurrent inhibition of ERK induces apoptosis [4] . Thus, the intensity, duration and balance of MAPK activities are important determinants of cell fate. The p38 MAPK signalling pathway also responds to pro-inflammatory cytokines such as interleukin (IL)-1β and tumour necrosis factor (TNF)-α, and controls immune responses by inducing the expression of effector cytokine genes [5] , [6] . As a result, the p38 pathway is an important target of anti-inflammatory drugs [7] . Cytokines induce rapid but transient activation of p38 (early phase), which then declines to a sustained low level that is only slightly higher than the pre-stimulation baseline (late phase). Nonetheless, the continued presence of activating cytokines is essential for proper induction of effector cytokines such as IL-6. Although it is believed that the duration and the temporal pattern of MAPK activation affect the quality of output signals [8] , [9] , [10] , the dynamics of p38 activity in the seemingly quiet late phase of cytokine activation are unknown. Here we report that, in this late phase, cells go through many cycles of p38 activation and inactivation, and that such p38 activity oscillation is important for efficient induction of its effector functions. FRET-based monitor of p38 MAPK activity We first examined the kinetics of IL-1β-induced p38 activation using conventional immunoblotting analyses. As previously shown, p38 is only transiently activated on stimulation of HeLa cells with IL-1β ( Fig. 1a ; within 1 h, early phase). However, if the p38 inhibitor was added after p38 activity had abated (at 2 h after IL-1β addition, late phase), IL-1β induction of IL-6 gene expression was severely suppressed ( Fig. 1b ), indicating that late-phase p38 activity, although very low, must be important for induction of its effector functions. As this low level p38 activity is unlikely to be sufficient to induce expression of p38-dependent pro-inflammatory genes, it is unclear why continuous presence of cytokine is necessary to do so. One possibility is that the p38 response of individual cells might differ from that of the average response of the cell population and thus a small number of cells with prolonged high activity of p38 might be masked by a large number of cells with low p38 activity. We therefore monitored p38 activity in individual living cells following cytokine stimulation. To do so, we developed a p38-specific kinase activity reporter based on the general design of previously reported MAPK reporters [10] , [11] , [12] , [13] , [14] ( Supplementary Fig. 1a ). Cells that stably express this p38 reporter (p38 reporter cells) were established using the PiggyBac transposon vector ( Supplementary Fig. 1b ). p38 reporter cells growing in a multi-well plate were analysed by placing under an automated fluorescence microscope equipped with a media circulation system. As expected, anisomycin, a potent activator of p38, induced strong Förster resonance energy transfer (FRET) signal (yellow fluorescent protein (YFP)/cyan fluorescent protein (CFP) ratio) from the probe-expressing cells ( Supplementary Fig. 1c , upper row). More important, the p38 inhibitor SB203580 suppressed the anisomycin-induced FRET signal at concentrations as low as 2 μM, which is unlikely to inhibit other kinases nonspecifically ( Supplementary Fig. 1c,d ). When p38α expression was inhibited by specific short interfering RNA (siRNA), FRET signal (induced by IL-1β) was suppressed to about 50% of the control cells ( Supplementary Fig. 1e ). The remaining FRET signal is likely due the uninhibited activity of p38β. Thus, we concluded that the obtained FRET signal was specific to the p38 family kinases. 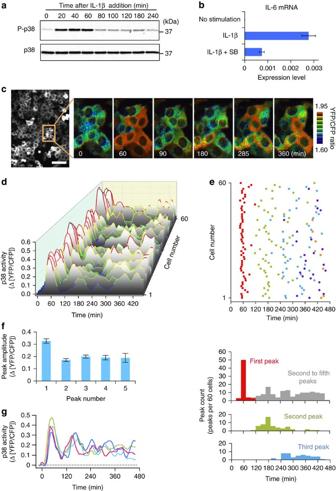Figure 1: Dynamics of p38 activation in individual cells. (a) Immunoblot analysis of p38 phosphorylation in HeLa cells. IL-1β (30 ng ml−1) was added at time=0. (b) HeLa cells were stimulated with IL-1β (30 ng ml−1) for 360 min and the IL-6 mRNA level was analysed using real-time quantitative PCR. The p38 inhibitor SB203580 (SB; 25 μM) was added at 120 min. Error bars represent s.e.m. (n=3). (c) Typical YFP/CFP ratio images showing p38 activation. HeLa cells stably expressing the p38 activity were stimulated continuously with IL-1β (10 ng ml−1). Scale bar, 40 μm. (d) Time-course of p38 activation in individual cells. HeLa cells were stimulated continuously with IL-1β (10 ng ml−1).n=60 cells. Colours as per scale bar inc. (e,f) Quantification of the peaks ind. (e) Peak times of consecutive rounds of p38 activity are indicated by dots of different colours (top panel). Histograms of peak times are shown below. Grey bars indicate the aggregate counts of the second through the fifth peaks.n=60 cells. (f) Mean amplitude of each p38 peak. Error bars represent s.e.m. (n=60, 56, 46, 24 and 7, respectively). (g) Overlay plot of typical p38 activity oscillations induced by continuous IL-1β stimulation (10 ng ml−1). Figure 1: Dynamics of p38 activation in individual cells. ( a ) Immunoblot analysis of p38 phosphorylation in HeLa cells. IL-1β (30 ng ml −1 ) was added at time=0. ( b ) HeLa cells were stimulated with IL-1β (30 ng ml −1 ) for 360 min and the IL-6 mRNA level was analysed using real-time quantitative PCR. The p38 inhibitor SB203580 (SB; 25 μM) was added at 120 min. Error bars represent s.e.m. ( n =3). ( c ) Typical YFP/CFP ratio images showing p38 activation. HeLa cells stably expressing the p38 activity were stimulated continuously with IL-1β (10 ng ml −1 ). Scale bar, 40 μm. ( d ) Time-course of p38 activation in individual cells. HeLa cells were stimulated continuously with IL-1β (10 ng ml −1 ). n =60 cells. Colours as per scale bar in c . ( e , f ) Quantification of the peaks in d . ( e ) Peak times of consecutive rounds of p38 activity are indicated by dots of different colours (top panel). Histograms of peak times are shown below. Grey bars indicate the aggregate counts of the second through the fifth peaks. n =60 cells. ( f ) Mean amplitude of each p38 peak. Error bars represent s.e.m. ( n =60, 56, 46, 24 and 7, respectively). ( g ) Overlay plot of typical p38 activity oscillations induced by continuous IL-1β stimulation (10 ng ml −1 ). Full size image Long-term oscillation of p38 activity When p38 reporter cells were stimulated over 60 min with various amounts of anisomycin, the intensity of the FRET signal increased homogenously among the cells in each population ( Supplementary Fig. 2a ). In contrast, IL-1β induced variable p38 activation within each population, especially at intermediate IL-1β doses ( ∼ 10 ng ml −1 ) ( Supplementary Fig. 2b ). When stimulated by higher doses of IL-1β (>10 ng ml −1 ), p38 activity reached a peak between 20 and 40 min but was on the decline by 60 min, which reflected the dynamics of p38 activation as analysed by immunoblotting analyses (see Fig. 1a ). Surprisingly, after p38 activity had completely subsided, it then started to increase again ( Fig. 1c ). Quantification of p38 activity in individual cells over time indicated that p38 activity oscillated, and that this oscillation continued with several peaks for at least 8 h ( Fig. 1d,e ). Mean amplitudes of the second and third peaks were 52% and 61%, respectively, of the initial peak ( Fig. 1f ). The first peaks displayed similar timing and amplitude for almost all cells, whereas the timing of the second and later peaks was more heterogeneous ( Fig. 1g ). Mean peak-to-peak intervals became gradually shorter in consecutive rounds: 148±9 min ( n =56) for first-to-second and 133±9 min ( n =46) for second-to-third intervals. When the responses were averaged over a cell population, p38 oscillatory dynamism was obscured and only the prominent first peak was observed ( Supplementary Fig. 3 ), consistent with immunoblotting analyses ( Fig. 1a ). To confirm that the oscillatory FRET signals are due to changing p38 activities in individual cells, we inhibited p38 activity by either 8 μM SB203580 or 1 μM BIRB796 ( Supplementary Fig. 4 ). When SB203580 or BIRB796 was added 30 min before the start of IL-1β stimulation, the FRET signal was completely suppressed (left panels). When SB203580 or BIRB796 was added 120 min after the addition of IL-1β, the first FRET peak was normal, but no subsequent peaks were observed (right panels). Therefore, we conclude that the oscillatory FRET signals in individual cells reliably report changing p38 activities. Negative feedback by MKP-1 induces oscillatory p38 activity Biochemical oscillation can be generated by certain network topologies, such as delayed negative-feedback loops [15] . To elucidate the properties of a putative feedback mechanism that might underlie p38 activity oscillation, we examined the input–output relationship following one or two pulsatile (6 min) IL-1β stimulations. On single pulse stimulation, there was only one transient p38 activation peak ( Fig. 2a ), suggesting that p38 activity oscillation requires the continued stimulation with IL-1β. When two IL-1β pulses were applied with a 60-min interval between them, the p38 activity response to the second stimulation was very weak, indicating that the p38 pathway had entered a refractory (or inhibited) state after the first strong response ( Fig. 2b , top panel). This inhibition was not due to downregulation of IL-1β-specific signalling, as p38 cannot be activated by a subsequent stimulation with TNF-α, which activates p38 via a different receptor ( Supplementary Fig. 5 ). However, the inhibition declined over time, as p38 activity in response to the second stimulation increased as the intervals between the first and second stimuli were lengthened ( Fig. 2b , middle and bottom panels). There was high variability in the amplitude of the second peak among individual cells ( Fig. 2c ). These results indicated that the inhibition of p38 activity lasted as long as 4 h after the initial stimulation, and that there was large variation in the rate of decline of this inhibition among individual cells. 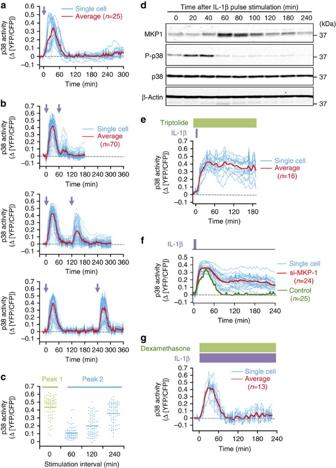Figure 2: Variation in the duration of p38 negative feedback regulation in individual cells. p38 responses to single pulse (a) or paired-pulse (b) IL-1β stimulation, with different intervals between the pulses. Times of the first and second stimulations are indicated by purple arrows. Reporter cells were stimulated with one or two 6-min IL-1β pulses (30 ng ml−1). Responses of individual reporter cells are shown by cyan curves and average traces are in red.n=25 foraand 70 for each panel inb. (c) Peak amplitude of the second peak at the indicated stimulation intervals.n=70 for each group. (d) Immunoblot analyses of the time course of p38 phosphorylation and MKP-1 expression in HeLa cells stimulated with a single 6-min IL-1β pulse (30 ng ml−1). (e–g) Effects of inhibiting or enhancing MKP-1 expression on p38 activation kinetics. Reporter cells were stimulated as indicated schematically above the graphs. Responses of individual reporter cells are shown by cyan curves and average traces are in red. (e) Effect of 30-min pretreatment with the MKP-1 inhibitor triptolide (3 μM) on p38 activation induced by a 6-min IL-1β pulse (30 ng ml−1). (f) Effect of inhibiting MKP-1 expression by specific siRNA on p38 activation induced by a 6-min IL-1β pulse (30 ng ml−1). The control curve (green) is the average of 25 siRNA-untreated cells shown ina. (g) Effect of the presence of the MKP-1 inducer dexamethasone (1 μM) on p38 activation induced by continuous IL-1β (30 ng ml−1) stimulation. Figure 2: Variation in the duration of p38 negative feedback regulation in individual cells. p38 responses to single pulse ( a ) or paired-pulse ( b ) IL-1β stimulation, with different intervals between the pulses. Times of the first and second stimulations are indicated by purple arrows. Reporter cells were stimulated with one or two 6-min IL-1β pulses (30 ng ml −1 ). Responses of individual reporter cells are shown by cyan curves and average traces are in red. n =25 for a and 70 for each panel in b . ( c ) Peak amplitude of the second peak at the indicated stimulation intervals. n =70 for each group. ( d ) Immunoblot analyses of the time course of p38 phosphorylation and MKP-1 expression in HeLa cells stimulated with a single 6-min IL-1β pulse (30 ng ml −1 ). ( e – g ) Effects of inhibiting or enhancing MKP-1 expression on p38 activation kinetics. Reporter cells were stimulated as indicated schematically above the graphs. Responses of individual reporter cells are shown by cyan curves and average traces are in red. ( e ) Effect of 30-min pretreatment with the MKP-1 inhibitor triptolide (3 μM) on p38 activation induced by a 6-min IL-1β pulse (30 ng ml −1 ). ( f ) Effect of inhibiting MKP-1 expression by specific siRNA on p38 activation induced by a 6-min IL-1β pulse (30 ng ml −1 ). The control curve (green) is the average of 25 siRNA-untreated cells shown in a . ( g ) Effect of the presence of the MKP-1 inducer dexamethasone (1 μM) on p38 activation induced by continuous IL-1β (30 ng ml −1 ) stimulation. Full size image Based on these properties, we suspected involvement of dual-specificity phosphatases, in particular of MKP-1/DUSP1, that can inactivate p38 by dephosphorylation [16] . A 6-min single-pulse of IL-1β stimulation induced MKP-1 expression that reached a maximum level at ∼ 60 min, followed by a gradual decline, whereas p38 phosphorylation decreased rapidly as MKP-1 accumulated ( Fig. 2d ). As expected, the p38 inhibitors SB203580 (ref. 17 ) and BIRB796 (ref. 18 ) suppressed MKP-1 induction at reasonably low concentration: 5 μM SB203580 and 0.1 μM BIRB796, respectively ( Supplementary Fig. 6a,b ). When cells were pre-treated with triptolide [19] , an inhibitor of MKP-1 expression ( Supplementary Fig. 6c ), a short pulsatile IL-1β stimulation induced sustained p38 activation ( Fig. 2e ). However, as triptolide affects the expression of many other genes as well as MKP-1 , we also inhibited MKP-1 expression using specific siRNA. When control cells were treated with a short pulsatile IL-1β stimulation, only transient p38 activation was observed ( Fig. 2f , green curve). In contrast, when cells transfected with MKP-1 siRNA were similarly treated, sustained p38 activation was observed ( Fig. 2f , red curve), indicating that MKP-1 is a major negative regulator of p38 activity. Dexamethasone is a good inducer of MKP-1 expression [20] . Indeed, simultaneous treatment of cells with IL-1β and dexamethasone induced much higher levels of MKP-1 than treatment with IL-1β alone ( Supplementary Fig. 6d ). Notably, when dexamethasone was added together with IL-1β, the second and the later oscillating p38 activity peaks were lost ( Fig. 2g ). Thus, we conclude that the negative feedback cycle between induction of MKP-1 expression by activated p38 and inhibition of p38 activity by MKP-1 governs oscillatory p38 activation. Mathematical modelling of oscillatory p38 activation To understand how the p38 activity oscillation arose, we constructed a mathematical model of the p38 feedback regulation ( Fig. 3a ; see Methods for detail). We estimated the rate constants of the component reactions based on experimental results and published data. When a constant stimulation was applied, the model generated oscillating p38 activation ( Fig. 3b ). Comparison of p38 activity (i.e., phosphorylated p38) and MKP-1 expression levels indicated that MKP-1 expression and p38 activation peaked alternately, and that new p38 cycles commenced when the MKP-1 concentration dropped to a threshold level. This model also recapitulated the results of paired pulse stimulation ( Supplementary Fig. 7a , compare with Fig. 2b ) as well as of pharmacological perturbation ( Supplementary Fig. 7b , compare with Fig. 2e,g ). By this model, it was demonstrated that oscillatory p38 activity arose from the delayed induction of MKP-1 expression by activated p38 as well as a slow degradation of MKP-1. 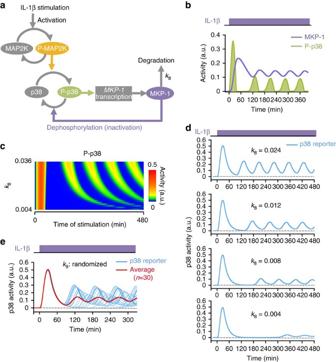Figure 3: A mathematical model of p38 activation that generates oscillatory dynamics. (a) A schematic diagram of p38 activation. (b) Calculated time course of p38 MAPK activity and MKP-1 expression under continuous IL-1β stimulation. a.u., arbitrary units. (c) Dependency of p38 activation dynamics on the degradation rate (k8) of MKP-1. Each horizontal line indicates a calculated time course of p38 activity (phospho-p38) with a differentk8(vertical axis) under conditions of continuous IL-β stimulation. Activity of p38 is as indicated by the color chart. (d,e) Predicted time courses of p38 reporter activity simulated under conditions of continuous IL-1β stimulation. For several fixedk8values (d) and for 30 randomizedk8values (e). Ine, individual traces are shown in cyan and the averaged trace is in red. Figure 3: A mathematical model of p38 activation that generates oscillatory dynamics. ( a ) A schematic diagram of p38 activation. ( b ) Calculated time course of p38 MAPK activity and MKP-1 expression under continuous IL-1β stimulation. a.u., arbitrary units. ( c ) Dependency of p38 activation dynamics on the degradation rate ( k 8 ) of MKP-1. Each horizontal line indicates a calculated time course of p38 activity (phospho-p38) with a different k 8 (vertical axis) under conditions of continuous IL-β stimulation. Activity of p38 is as indicated by the color chart. ( d , e ) Predicted time courses of p38 reporter activity simulated under conditions of continuous IL-1β stimulation. For several fixed k 8 values ( d ) and for 30 randomized k 8 values ( e ). In e , individual traces are shown in cyan and the averaged trace is in red. Full size image In the paired-pulse experiments with intervals of 120 or 240 min between pulses, the amplitude of the second response, a measure of the strength of negative feedback, was highly variable ( Fig. 2b,c ). This finding suggested that the degradation rate of MKP-1 ( k 8 ; see Fig. 3a ) might be heterogeneous within a population. The simulation results of paired-pulse stimulations with varied k 8 values matched well with the experimental results in that the amplitude of the second p38 activity peak was highly sensitive to k 8 change for 120- and 240-min intervals, but not for 60-min intervals ( Supplementary Fig. 7c ). When the response to a continuous stimulation was simulated using different k 8 values, the second p38 activity peak was significantly delayed and weakened, as k 8 became smaller, whereas the first p38 activity peak was essentially unaffected ( Fig. 3c,d ). Averaging of simulated p38 traces with varied k 8 values resulted in a robust first peak that was followed by low sustained activity ( Fig. 3e ), which recreated the actual experimental results. It has been reported that the stability of MKP-1 is variable, owing to posttranslational modifications [21] . Thus, one possible cause of asynchrony in the p38 oscillation is cell-to-cell variability of MKP-1 degradation rate. p38 oscillation influences pro-inflammatory gene expression We next investigated whether oscillation of p38 activity plays a role in induction of the pro-inflammatory genes. For that purpose, we applied different temporal patterns of IL-1β stimulation to the HeLa cells ( Fig. 4a , protocol numbers 1–6). Robust messenger RNA expression of the IL-6 , IL-8 and COX-2 genes was induced by continuous IL-1β stimulation for 6 h ( Fig. 4b ; number 2 protocol). As expected, their expression was suppressed by the p38 inhibitor SB203580 (25 μM) (number 3 protocol). The residual gene expression is probably due to non-p38 signalling induced by IL-1β (ref. 22 ). Addition of 25 μM SB203580 at 2 h, when the initial p38 activation had already subsided (number 4 protocol), did not increase the expression of these genes at 6 h. Lower concentration of SB203580 (8 μM) or another p38-inhibitor BIRB796 (1 μM) had the same effect as 25 μM SB203580 ( Supplementary Fig. 8 ). Consistent with the protocol 4 experiments, a single transient (6 min) IL-1β stimulation, which generated a robust, but single, p38 peak (number 5 protocol), failed to maintain the expression of these genes at 6 h. We found, however, that the continuous presence of IL-1β was unnecessary for efficient gene expression, as repetitive short pulse stimulations (6 min at 60-min intervals) (number 6 protocol) attained gene expression levels equal to or even higher than the continuous IL-1β stimulation. 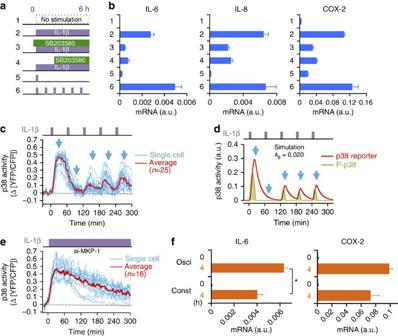Figure 4: Oscillation of p38 activity regulates expression of pro-inflammatory genes. (a) Diagrams of stimulation/inhibition protocols. HeLa cells were left unstimulated or were stimulated with IL-1β (30 ng ml−1) continuously for 6 h, or with single or multiple 6 min pulses as indicated. SB203580 was added 30 min before (number 3) or 2 h after (number 4) IL-1β addition. (b) The mRNA expression of pro-inflammatory genes was determined at the end of the 6-h stimulation protocols using real-time quantitative PCR. Error bars represent s.e.m. (n=3). (c) Time course of p38 activation induced by five successive IL-1β pulses (30 ng ml−1, 6 min per pulse with 60-min intervals between pulses) was examined by p38 FRET imaging. Cyan lines indicate individual cell traces and the red line indicates the averaged trace (n=25 cells). (d) Simulation of phospho-p38 (green) and p38 reporter activity (red) under the same conditions as inc. (e) Time course of p38 activation induced by constant IL-1β stimulation (30 ng ml−1) in reporter cells treated with siRNA targeting endogenous MKP-1 (si-MKP-1) was examined by p38 FRET imaging. Cyan and red lines are as inc(n=16 cells). (f) Expression of pro-inflammatory cytokine mRNA in HeLa cells in which p38 activity oscillates (stimulation conditions as inc) or p38 activity is nearly constant (stimulation conditions as ine). Amount of mRNA was quantified by quantitative PCR at 4 h. Error bars represent s.e.m. (n=3). *P=0.014, Student’st-test. Figure 4: Oscillation of p38 activity regulates expression of pro-inflammatory genes. ( a ) Diagrams of stimulation/inhibition protocols. HeLa cells were left unstimulated or were stimulated with IL-1β (30 ng ml −1 ) continuously for 6 h, or with single or multiple 6 min pulses as indicated. SB203580 was added 30 min before (number 3) or 2 h after (number 4) IL-1β addition. ( b ) The mRNA expression of pro-inflammatory genes was determined at the end of the 6-h stimulation protocols using real-time quantitative PCR. Error bars represent s.e.m. ( n =3). ( c ) Time course of p38 activation induced by five successive IL-1β pulses (30 ng ml −1 , 6 min per pulse with 60-min intervals between pulses) was examined by p38 FRET imaging. Cyan lines indicate individual cell traces and the red line indicates the averaged trace ( n =25 cells). ( d ) Simulation of phospho-p38 (green) and p38 reporter activity (red) under the same conditions as in c . ( e ) Time course of p38 activation induced by constant IL-1β stimulation (30 ng ml −1 ) in reporter cells treated with siRNA targeting endogenous MKP-1 (si-MKP-1) was examined by p38 FRET imaging. Cyan and red lines are as in c ( n =16 cells). ( f ) Expression of pro-inflammatory cytokine mRNA in HeLa cells in which p38 activity oscillates (stimulation conditions as in c ) or p38 activity is nearly constant (stimulation conditions as in e ). Amount of mRNA was quantified by quantitative PCR at 4 h. Error bars represent s.e.m. ( n =3). * P =0.014, Student’s t -test. Full size image We thus examined the temporal pattern of p38 activation in cells under the number 6 stimulation protocol. Experimentally, a regimen of five repetitive pulsatile stimulations induced four peaks of p38 activity; the second pulse failed to induce p38 activation ( Fig. 4c ). The mathematical model very accurately recapitulated these complex dynamics of p38 activation induced by discontinuous IL-1β stimulation ( Fig. 4d shows the average response, whereas Supplementary Fig. 9 shows the responses in individual cells). Thus, repetitive pulsatile IL-1β stimulation generated p38 activation time course that was similar to the oscillatory p38 activation generated by the continuous presence of IL-1β, although the former was more synchronous than the latter. More detailed analyses of gene expression time courses demonstrated that a single p38 activity peak (generated by a single 6 min IL-1β stimulation; number 5 protocol in Fig. 4a ) rapidly induced expression of the pro-inflammatory genes that lasted only short period of time ( Supplementary Fig. 10a , red curves). In contrast, repetitive activation of p38 (generated by repetitive pulsatile IL-1β stimulations; number 6 protocol in Fig. 4a ) maintained high gene expression levels over an extended period ( Supplementary Fig. 10a , green curves). These differences were not unexpected, because the cumulative p38 activity was much higher in the second regimen (compare Figs 2a and 4c ). We then compared gene expression levels between cells in which p38 was intermittently activated (as in Fig. 4c ) and cells in which p38 was continuously activated without oscillation. To create the latter condition, we knocked down MKP-1 expression by specific siRNA and stimulated the cells with continuous IL-1β exposure ( Fig. 4e ). In these cells, IL-1β stimulation induced sustained (although gradually declining) p38 activity for at least 5 h. By comparing Fig. 4c,e , it is obvious that the cumulative p38 activity is much higher in the latter cells. Nevertheless, mRNA levels of pro-inflammatory genes were similar or even higher in cells in which p38 was intermittently activated than in cells in which p38 was continuously active ( Fig. 4f and Supplementary Fig. 10b ). Thus, we conclude that oscillatory p38 activity induces pro-inflammatory genes more efficiently than non-oscillatory continuous p38 activity. Finally, we examined the optimal time interval of p38 oscillation that induces efficient pro-inflammatory gene expression. For this purpose, cells were stimulated with 6 min IL-1β pulses at different (60, 100, 150 and 300 min) intervals ( Supplementary Fig. 10c ). Most efficient expression of the IL-6 and IL-8 genes was observed when cells were repetitively stimulated with either 60- or 100-min interval, whereas the COX-2 gene was expressed most efficiently when stimulated with 60-min interval ( Supplementary Fig. 10d ). It is interesting to note that these intervals coincide with those of the intrinsic p38 oscillation induced by constant IL-1β stimulation (see Fig. 1g ). We found that constant IL-1β stimulation induces oscillation of p38 MAPK activity. The activity of other MAPKs is also known to oscillate but through different mechanisms. In yeast, the mating pheromone-responsive Fus3 MAPK undergoes sustained oscillation of its phosphorylation and activation, which lasts for at least 8 h with three separate peaks [23] . This oscillation requires the negative regulator of G-protein signalling Sst2, and also partially requires the MAPK phosphatase Msg5. Fus3 oscillation can be detected by immunoblotting analyses, because its oscillation is synchronous. However, in other cases, such as in the present study, oscillation is asynchronous and can be detected only when the response of individual cells are studied. In mammalian cells, rapid nuclear-cytoplasmic shuttling of the ERK MAPK with a rapid periodicity of ∼ 15 min is induced by epidermal growth factor [24] . Much faster oscillation of ERK in the Shankaran study is distinct from that of p38 oscillation, in which periodicity is longer than 2 h. More recently, using a FRET-based ERK activity reporter, Aoki et al . [12] reported that ERK activity oscillates with much longer periodicity. This ERK activity oscillation is generated mainly by stochastic and autonomous excitation of the Raf MAPKKK in the absence of external stimulation and is also different from the mechanism of p38 oscillation that depends on external stimulation. In another study, also using a FRET-based ERK activity reporter, Albeck et al . [25] reported that, under steady-state conditions, ERK activity oscillates asynchronously with periodicity that is determined by the concentration of external epidermal growth factor. Finally, Regot et al . [26] also showed that JNK and ERK (but not p38) activities fluctuate in living cells, by employing multiple kinase activity reporters based on phosphorylation-induced nuclear translocation. Although they did not explore the role of phosphatases in the JNK/ERK activity oscillation, Albeck’s and Regot’s findings might be mechanistically related to our finding that a negative feedback loop involving the MKP-1 phosphatase is important for the p38 activity oscillation. Thus, oscillation of MAPK activity is more commonplace than previously thought, but in most cases their oscillations are observable only when individual cells are studied. Oscillatory p38 activation probably satisfies conflicting demands on the p38 pathway. Thus, for proper immune responses, it is important that the target cells continuously respond to the presence of IL-1β or TNF-α through the expression of effector genes. However, although continuous activation of p38 may achieve this goal, it could potentially be deleterious to the cell and may even induce apoptosis [27] . Oscillatory p38 activation therefore may ensure that sufficient expression of effector genes occurs without causing cellular damage. Indeed, we found that oscillatory p38 activation induces the same or even higher levels of the target gene expression than the constant p38 activity induces, in spite of the fact that the cumulative p38 activity is much less in the former case. An asynchronous p38 oscillation may be important, as a synchronous p38 activity oscillation would lead to periodic and steep rises of effector cytokine expression, which might in turn be damaging to the immune system. Therefore, the asynchronous activation of p38 among cells would ensure that a constant expression level of effector genes is maintained at the population level, without causing damage. In contrast, the synchronous activation of the yeast Fus3 MAPK may be important to ensure that all the cells in a population become mating-competent simultaneously. Thus, although various MAPK pathways employ similar sets of signalling components, they are configured differently to suit specific requirements. Quantitative analyses of mathematical models are important means to understand the complex interplays among intracellular signalling pathways. To model a signalling pathway mathematically, it is essential to obtain quantitative values for key activities in the pathway. However, the current study as well as others has clearly demonstrated that population level measurements of these values are inadequate in many instances, as the dynamic behaviour of individual cells is totally lost in the population average. Therefore, it is essential to obtain quantitative measurements of these values in individual cells. FRET-based activity reporters are very useful for such measurements. In conclusion, constant cytokine stimulation generates an oscillatory activation of p38 MAPK that is important for efficient induction of pro-inflammatory gene expression. p38 activity oscillation allows cells to respond optimally to continuous cytokine stimulation such as occurs during infection, while preventing cell damage and apoptosis that can be caused by continuous and excessive p38 activation [4] . These findings should be relevant to the development of safer and more effective anti-inflammatory therapeutics. Construction of p38 MAPK activity reporters p38 MAPK activity reporters were constructed using the pCAGGS-based vector pYL225 (ref. 14 ), which contains the open reading frames of the enhanced YFP YPet and the super-enhanced CFP. The most efficient reporter so far constructed, termed ‘PerKy-38’, is composed of the following segments (from the N terminus to the carboxy terminus): YPet (amino acid residues 1–228), Linker 1 (Leu-Glu), the WW domain of Pin1 (amino acid residues 1–54), Linker 2 (Ala-Ser), the p38-docking domain of Mef2A (amino acid residues 266–291), the c-Jun MAPK phosphorylation region excluding the JNK docking site (amino acid residues 54–73), Linker 3 (Gly-Gly-Arg-Gly-Gly) and super-enhanced CFP (amino acid residues 1–237). The nuclear export signal of MEK1 was added at the 3′-end of the reporter, as the reporter without nuclear export signal tended to accumulate in the nucleus. The DNA segment encoding the Pin1 WW domain was amplified by PCR using a Pin1-encoding plasmid as a template. The DNA segments encoding the Mef2A and c-Jun fragments were prepared by using synthetic oligonucleotides. Cell lines Cell lines that constitutively express the PerKy-38 reporter were established using the PiggyBac expression system (System Biosciences, Inc.). The coding sequence of the p38 reporter was inserted between the EcoRI and BamHI cloning sites of the donor plasmid PB510B-1 (PB-CMV-MCS-EF1-Puro). HeLa cells were co-transfected with the donor plasmid for the p38 reporter and the expression plasmid for the PiggyBac transposase. Transfection was carried out using Effectene (Qiagen) in accordance with the manufacturer’s standard protocol. Cells that had integrated the p38 reporter into chromosomal locations, and stably express the p38 reporter, were selected using puromycin. Cell culture and transfection HeLa cells were maintained in DMEM medium supplemented with 10% fetal bovine serum (FBS), L -glutamine, penicillin and streptomycin. For imaging analyses, cells stably expressing the p38 reporter were plated, a day before imaging analysis, on a 24-well glass-bottom plate (Iwaki, 5826-024) or on a 35-mm-diameter glass-bottom dish (Iwaki, 3910-035) at 30% confluency. Time-lapse imaging For time-lapse analyses, cells were starved in Medium 199 (Gibco, 11043-023) supplemented with 0.5% FBS for at least 8 h before imaging. All imaging analyses were carried out at 37°C under 5% CO 2 . Fluorescence images of the cells were captured using the Nikon TE-2000E inverted microscope equipped with the CFI PlanApoVC × 20 (numerical aperture 0.75) objective, a CoolSnapHQ CCD (charge-coupled device) camera (Roper), a heat-CO 2 chamber, a mercury lamp (Nikon) and a computer-controlled emission filter changer (Ludl Electronic Products). A FRET filter set (Semrock) was used to excite the fluorescent proteins at 440 nm, and to acquire fluorescence images at 480 nm (for CFP) and at 535 nm (for YFP). Pixel-by-pixel YFP/CFP ratio images were generated using the MetaMorph software (Molecular Device) and were displayed with an intensity modulated display mode based on the YFP fluorescence intensity. Cells were stimulated by rapidly substituting the bathing medium with stimulation medium containing IL-1β or anisomycin using a media circulation pump (ATTO, AC-2120). Immunoblotting Cells were plated, a day before analysis, onto a 6-well plate (Falcon, 353046) at 30% confluency. Cells were starved in Medium 199 containing 0.5% FBS for 8 h before stimulation with IL-1β (30 ng ml −1 ). Immediately after stimulation, the cells were washed twice with ice-cold PBS solution and lysed directly in SDS sample buffer (65 mM Tris-HCl pH 6.8, 5% 2-mercaptoethanol, 3% SDS, 0.0025% bromophenol blue and 10% glycerol). Samples were then boiled for 5 min, separated by SDS–PAGE (10% poly acrylamide gel), transferred onto a nitrocellulose membrane and immunoblotted with antibodies. Anti-p38 (Santa Cruz sc-535 at 1:1,000 dilution) and anti-phospho-p38 (Cell Signaling Technology 9211S at 1:1,000 dilution) were used for detection of the phosphorylation status of endogenous p38 protein in HeLa cells. Anti-MKP-1 (Santa Cruz sc-370 at 1:250 dilution) was used to detect MKP-1 protein expression. Anti-β-actin (Cell Signaling 4967S at 1:1,000 dilution) was used for a loading control. Digital images were captured using the ChemiDoc XRS+ system (Bio-Rad). Full scans of representative immunoblots are presented in Supplementary Fig. 11 . mRNA expression analyses Endogenous mRNA expression level was analysed using a two-step real-time quantitative PCR method. Cells were starved and stimulated as described for immunoblotting, and cellular RNA was purified using RNeasy Mini (Qiagen) according to the manufacturer’s protocol. Reverse transcription of mRNA was performed using PrimeScript reverse transcriptase (Takara), then DNA was analysed using real-time PCR thermal cycler system (Takara, TP800) in the presence of SYBR Green I/ ExTaqII polymerase (Takara, RR820A). The expression level of the target mRNA relative to that of the GAPDH mRNA was determined using a standard comparative C T method. Three independent samples were analysed for each condition. The nucleotide sequences of PCR primers are as follows: GAPDH forward (Fw) 5′-GCACCGTCAAGGCTGAGAAC-3′, GAPDH reverse (Rv) 5′-TGGTGAAGACGCCAGTGGA-3′; IL-6 Fw 5′-GCCAGAGCTGTGCAGATGAG-3′, IL-6 Rv 5′-TCAGCAGGCTGGCATTTG-3′; IL-8 Fw 5′-GTGCAGAGGGTTGTGGAGAAGTTT-3′, IL-8 Rv 5′-ACCAGGAATCTTGTATTGCATCTGG-3′; COX-2 Fw 5′-TGAAACCCACTCCAAACACAG-3′, COX-2 Rv 5′-TCAGCATTGTAAGTTGGTGGAC-3′. Primer sets were obtained from Takara (GAPDH: HA067812, IL-6: HA209655, IL-8: HA217928 and COX-2: HA209441). siRNA experiments p38 reporter cells were transfected with siRNAs using Lipofectamine RNAiMAX (Invitrogen) according to the manufacturer’s protocol. Expression of p38α/MAPK14 was inhibited by a mixture of two siRNA sequences (catalogue numbers 18464 and 18465, Sigma-Aldrich), whereas the MKP-1-specific siRNA (catalogue number GS1843, Qiagen) contained four siRNA sequences. Negative control siRNA (S5C-0600) was purchased from Cosmo Bio (Tokyo). Transfected cells were subjected to imaging analysis 48 h after transfection. Mathematical modelling and simulation The model consists of the following set of differential equations. Implementation of the model and calculation were done using the Mathematica programme (Wolfram Research). Equations: (i) Activation of MAP2Ks that activate p38. (ii) Activation and inactivation of p38 MAPK. (iii) Transcription of the MKP-1 mRNA. (iv) Protein expression of MKP-1 (v) Conversion of p38 activity to the p38 FRET reporter signal. Following equations were used for simulating the effect of pharmacological inhibitors. (vi) Modification of equation (iii) in the presence of dexamethasone. (vii) Modification of equation (iv) in the presence of triptolide. The kinetics of p38 inactivation by MKP-1 was expressed based on Michaelis–Menten equation, which was obtained by means of quasi-steady-state approximation (equation (ii)). In the model, a delay in MKP-1 expression relative to p38 activation, which was evident from our experimental data, was introduced by introduction of a rate-limiting step of MKP-1 transcription in equation (iii). Variables: MAP2K[ t ], the activity of the MAP2Ks that activate p38. MAPK[ t ], the activity of the p38 MAPK. MKP1RNA[ t ], the MKP-1 gene transcription level. MKP1[ t ], the MKP-1 protein expression level. S[ t ], the stimulatory input. FRET[ t ], the signal of FRET reporter. S[ t ] was set to 0 when there is no stimulation and 1 when stimulated. Parameters: k 0 , the rate constant for MAP2K activation (0.06 min −1 ). k 1 , the rate constant for MAP2K deactivation (0.15 min −1 ). k 2 , the rate constant for p38 MAPK activation (0.15 min −1 ). k 3 , the maximum reaction rate of p38 MAPK inactivation by MKP-1 (0.16 min −1 ). k 4 , an equivalent of the Michaelis–Menten constant for the reaction of MKP-1-mediated p38 inactivation (0.0001). k 5 , the rate constant for MKP-1 gene transcription (0.055 min −1 ). k 6 , the rate constant for degradation of MKP-1 gene transcript (0.05 min −1 ). k 7 , the rate constant for MKP-1 protein expression (0.20 min −1 ). k 8 , the rate constant for MKP-1 protein degradation (0.02 min −1 ). k 9 , the rate constant for FRET reporter activation by active p38 MAPK (0.2 min −1 ). k 10 , the rate constant for FRET reporter inactivation (0.05 min −1 ). k 11 , the rate constant for MKP-1 protein expression in the presence of triptolide (0.0002, min −1 ). k 12 , the rate constant for MKP-1 gene transcription induced by dexamethasone treatment (0.003 min −1 ). How to cite this article: Tomida, T. et al . Oscillation of p38 activity controls efficient pro-inflammatory gene expression. Nat. Commun. 6:8350 doi: 10.1038/ncomms9350 (2015).